Laser-induced ultrafast demagnetization in the presence of a nanoscale magnetic domain network Femtosecond magnetization phenomena have been challenging our understanding for over a decade. Most experiments have relied on infrared femtosecond lasers, limiting the spatial resolution to a few micrometres. With the advent of femtosecond X-ray sources, nanometric resolution can now be reached, which matches key length scales in femtomagnetism such as the travelling length of excited 'hot' electrons on a femtosecond timescale. Here we study laser-induced ultrafast demagnetization in [Co/Pd] 30 multilayer films, which, for the first time, achieves a spatial resolution better than 100 nm by using femtosecond soft X-ray pulses. This allows us to follow the femtosecond demagnetization process in a magnetic system consisting of alternating nanometric domains of opposite magnetization. No modification of the magnetic structure is observed, but, in comparison with uniformly magnetized systems of similar composition, we find a significantly faster demagnetization time. We argue that this may be caused by direct transfer of spin angular momentum between neighbouring domains. The phenomenon of ultrafast demagnetization [1] , first discovered in 1996, resulting from excitation by an intense femtosecond infrared laser pulse, has been extensively investigated, yet its underlying mechanism remains poorly understood [2] . Additionally, it has attracted considerable interest as a possible path to magnetization control on a femtosecond timescale [3] . Most commonly, the magneto-optical Kerr effect (MOKE) is exploited as a femtosecond probe of the temporal evolution of magnetization [2] . Despite some controversy about the validity of MOKE as a probe of the magnetization of an excited system on the femtosecond timescale [4] , [5] , [6] , [7] , significant progress has been made: the importance of subtle effects, such as direct transfer of spin angular momentum [8] or coherent magneto-optical processes [9] , have been revealed. Phenomenological and microscopic models have been proposed and further refined [10] , [11] , [12] , [13] . However, up to now, ultrafast demagnetization has not been studied at the magnetic domain level itself, owing to the spatial resolution limit set by the infrared laser wavelength of the MOKE probe pulse. Intuitively, this can be seen as one of the limitations of the available experimental data, because the particularities of an underlying magnetic domain structure can have an influence on macroscopic properties of a ferromagnetic material. Moreover, nanometre distances are the relevant length scale for energy and angular momentum transfer occurring on the femtosecond timescale between electrons, spins and the lattice, which are the processes underlying the macroscopically observed ultrafast demagnetization phenomenon. X-rays, with their wavelength of a few nanometres or shorter, potentially offer nanometre spatial resolution in time-resolved experiments. In this regard, the recent advent of femtosecond-pulsed soft and hard X-ray sources in the form of free-electron lasers [14] , [15] (XFELs), synchrotron radiation femtoslicing [16] , [17] and high-order harmonic generation (HHG) [18] sources, has opened up the possibility of novel experiments, which combine, for the first time, femtosecond temporal and nanometre spatial resolution in an element-specific observation of ultrafast dynamics occurring in complex materials. The first time-resolved experiments relying on femtosecond X-ray sources have already led to new insight into ultrafast magnetization dynamics [19] , [20] , [21] , [22] . Snapshot imaging of nanoscale magnetic structures using a single femtosecond XFEL pulse has also been demonstrated [23] , [24] . However, the full potential of these new sources, combining temporal and spatial resolution, had not been exploited so far. This gap is filled by our study on laser-driven demagnetization in a [Co/Pd] 30 multilayer having a nanometric magnetic domain structure. This work fully exploits the capabilities of HHG femtosecond soft X-ray sources by combining, in an infrared pump–X-ray probe experiment, a temporal resolution of about 40 fs with sub-100 nm spatial resolution. Our experiment reveals that locally, within each magnetic domain, the magnetization undergoes a rapid decrease, on the femtosecond timescale, as previously observed macroscopically for uniformly magnetized thin films. The overall magnetic domain structure, on the other hand, retains its organization, even for the highest excitation power accessible in this experiment. Surprisingly, the observed demagnetization times (~100 fs) are shorter than those reported for uniformly magnetized Co compounds. Furthermore, they do not vary with excitation power as suggested by previous work. We postulate that these observations are a consequence of direct transfer of spin angular momentum between neighbouring domains. 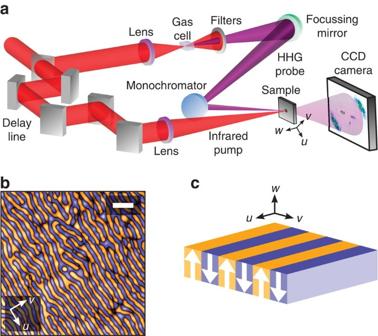Figure 1: Set-up and sample characteristics. (a) Schematic diagram of the pump–probe set-up. (b) Magnetic force micrograph of the magnetic structure of the sample, a [Co−Pd]30multilayer film. The white scale bar represents 500 nm. (c) This structure consists of alternating up-and-down magnetic domains aligned along the same direction with an out-of-plane magnetization (white arrows). Experimental details Figure 1a is a schematic representation of the set-up. The static part of the experiment (without infrared pump) has been described in more detail in refs 25 , 26 . In short, femtosecond harmonic pulses are generated in a gas cell, monochromatized at an energy of 60 eV (20.7nm) and focussed onto the sample. This photon energy matches the Co M 3 absorption edge, which exhibits a pronounced resonant magneto-optical effect [27] . As demonstrated previously [26] , [28] , this gives rise to magnetic scattering even when using linearly polarized harmonics. A small fraction of the infrared laser beam driving the HHG process is used as a pump initiating the demagnetization dynamics. Because pump and probe pulses originate from the same laser pulse, this set-up is inherently jitter free. This allows us to follow the demagnetization dynamics with a time resolution of about 40 fs (see Methods ), which is significantly better than what has been achieved so far in pump-probe experiments at femtoslicing and XFEL sources [19] , [20] . Figure 1: Set-up and sample characteristics. ( a ) Schematic diagram of the pump–probe set-up. ( b ) Magnetic force micrograph of the magnetic structure of the sample, a [Co−Pd] 30 multilayer film. The white scale bar represents 500 nm. ( c ) This structure consists of alternating up-and-down magnetic domains aligned along the same direction with an out-of-plane magnetization (white arrows). Full size image The sample used was a 30nm thin [Co(0.4 nm)/Pd(0.6 nm)] 30 multilayer film, deposited by magnetron sputtering on a silicon nitride membrane, which exhibits an out-of-plane magnetic anisotropy ( Supplementary Fig. S1 ). A demagnetization procedure was applied [29] to prepare a magnetic domain structure of aligned stripes ( Fig. 1b,c ). This acts as a diffraction grating for the resonant soft X-rays [26] , giving rise to plus-and-minus first-order diffraction peaks as shown in Fig. 2a . The intensity, I ( q ), of this resonant elastic magnetic scattering pattern, recorded with an in-vacuum charge-coupled device (CCD) camera, is proportional to | S ( q )| 2 with q the wave vector transfer and S ( q ) the Fourier transform of the magnetic domain structure [23] . The temporal evolution of the scattering pattern thus reveals the evolution of the magnetic domain structure on the nanometre length scale during the demagnetization process. The achievable spatial resolution is in principle only limited by the wavelength employed, and magnetic domains as small as 60 nm are easily detected in our set-up [26] . Moreover, the integrated diffracted intensity in the first-order peaks is proportional to T and M 2 , where T is the average transmission of the sample and M the magnetization magnitude within each magnetic domain (Equation (3) and (4)). The film average transmission being constant during the experiment ( Supplementary Fig. S2 ), the magnetization at the magnetic domain level can be retrieved for each delay. We note that in our experiment, the integrated magnetization along the film normal is measured, treating each depth of the film on an equal footing. This is contrary to an optical MOKE experiment, where the sampling depth is set by the penetration of the optical light (15 nm in metallic films). 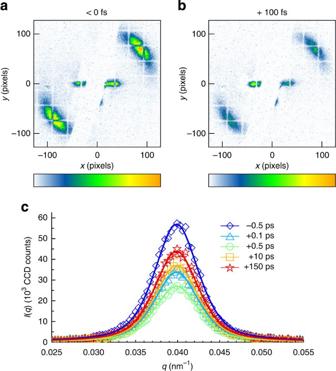Figure 2: Resonant magnetic scattering patterns and radial integration of the intensity. (a,b) The resonant magnetic scattering patterns exhibit two well-defined bright spots indicating that the magnetic structure of the sample consists of aligned magnetic domains (the scale bars go from 0, white, to 750 CCD counts, orange; 16 CCD counts ~1 detected photon). Whereas the overall pattern remains the same for negative, panel (a), and positive, panel (b), delays, a clear decrease of the integrated intensity can be observed a few hundreds of femtosecond after an optical excitation. (c) Scattered intensity as a function of wave-vector transfer,q, for increasing time delays for a pump fluence of 7.5mJcm−2. The solid lines are fits by the same pseudo-Voigt profile scaled to take into account the evolution of the integrated intensity. The curves exhibit one peak centre atq0=0.04nm−1 with an FWHM, Δq0, of 0.006nm−1 corresponding to a mean magnetic domain width of about 80 nm. The high signal-to-noise ratio of these curves yields a very sensitive probe for the occurrence of spatial variations of the magnetic domain structure during the ultrafast demagnetization process. Figure 2: Resonant magnetic scattering patterns and radial integration of the intensity. ( a , b ) The resonant magnetic scattering patterns exhibit two well-defined bright spots indicating that the magnetic structure of the sample consists of aligned magnetic domains (the scale bars go from 0, white, to 750 CCD counts, orange; 16 CCD counts ~1 detected photon). Whereas the overall pattern remains the same for negative, panel ( a ), and positive, panel ( b ), delays, a clear decrease of the integrated intensity can be observed a few hundreds of femtosecond after an optical excitation. ( c ) Scattered intensity as a function of wave-vector transfer, q , for increasing time delays for a pump fluence of 7.5mJcm−2. The solid lines are fits by the same pseudo-Voigt profile scaled to take into account the evolution of the integrated intensity. The curves exhibit one peak centre at q 0 =0.04nm−1 with an FWHM, Δ q 0 , of 0.006nm−1 corresponding to a mean magnetic domain width of about 80 nm. The high signal-to-noise ratio of these curves yields a very sensitive probe for the occurrence of spatial variations of the magnetic domain structure during the ultrafast demagnetization process. Full size image Analysis of time-resolved magnetic scattering patterns Typical scattering patterns (accumulated over 500 s and covering the q -range from 0.01 to 0.12nm −1 ) obtained at a pump fluence of 7.5mJcm−2 and reproduced in Fig. 2a,b , show clearly the plus-and-minus first order of the magnetic domain grating. As the diffraction efficiency is very small (~10 −6 ) [26] , a beamstop has to be used to prevent the direct beam from saturating the CCD camera. The two patterns have been recorded for negative ( Fig. 2a ) and positive ( Fig. 2b ) time delays of the X-ray probe pulse with respect to the infrared pump pulse. Whereas the overall structure of the two patterns is the same, the decrease in intensity of the diffraction peaks is evident to notice only 100 fs after the infrared pump pulse has been applied. We note that the general structure of the magnetic scattering pattern does not change in this repetitive pump-probe experiment. This suggests that the overall magnetic domain structure recovers after each pump-probe cycle, at least within the statistical description underlying the observed scattering pattern [29] . To obtain a detailed view on the spatial evolution of the magnetic domain structure during the demagnetization process, we perform radial and azimuthal integration of the scattering pattern I ( q ). In Fig. 2c , radial intensity profiles are plotted for different pump-probe time delays. The relation between real space distances, and wave vector transfer, q , is given by equation (1). A comparison of these curves reveals that peak position and shape remain unchanged. In particular, independently of the applied pump-probe delay, one does not observe any additional scattering at higher q values, which would correspond to breaking-up of magnetic domains in smaller ones. An absence of any variations with pump-probe delay is also observed when comparing the azimuthal integrals of I ( q ) ( Supplementary Fig. S3 ), which indicates that the alignment of the magnetic domains remains unchanged. We can thus conclude that the magnetic stripe domain pattern does remain unchanged during the demagnetization process, with a mean domain width of 2 π / q 0 (~80nm) and an in-plane correlation length of 2 π /Δ q 0 (~1μm). The evolution of the local magnetization amplitude is revealed by the peak intensity of the radial integrals shown in Fig. 2c . It reproduces the general behaviour previously observed for transition metal-based ferromagnetic materials [2] , namely, a very fast initial demagnetization on the timescale of a few hundred femtoseconds followed by a slow partial recovery. This behaviour is described by the phenomenological three temperature model proposed for uniformly magnetized films [1] . The electronic system is heated by the optical excitation almost instantaneously. Its energy is rapidly transferred to the spin system causing the initial rapid demagnetization. The subsequent thermalization of the electron and spin system with the lattice results in a partial recovery of the magnetization. On a longer timescale (a few nanoseconds), the three subsystems cool down because of heat transfer to the surrounding material, and the magnetization recovers completely. How exactly these processes occur at the microscopic level is still actively debated [2] , [13] . In our experiment, the initial heating of the spin system seems to be very fast, because within the first 100 fs, more than two-thirds of the magnetic scattering signal is lost. 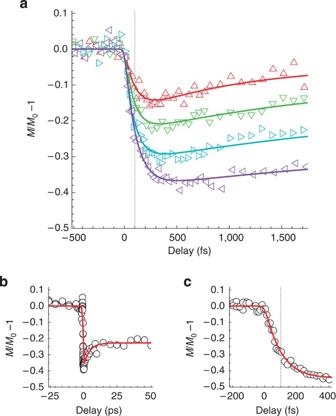Figure 3: Magnetization as a function of time delay for the [Co−Pd]30 multilayer film. (a) Demagnetization curves obtained for different pump fluences: 4, 6, 7.5 and 9 mJ cm−2(respectively; red, up; green, down; cyan, right; and purple, left triangles). The probe fluence, 5×10−5mJ cm−2, is negligible compared with the pump fluence26. The solid lines represent the best fits obtained for each fluence. The characteristic thermalization times,τth, found are all between 90 and 110 fs with an error of ±25 fs. No clear relation between the pump fluence andτthhas been observed. (b) Example of a long delay scan used to determine the spin-phonon relaxation constant,τs−ph. Long delay scans have been performed for each fluence. (c) High-resolution demagnetization curve obtained for the highest possible pump fluence (11 mJ cm−2), yielding a demagnetization of 44% and clearly showing a thermalization time of ~100 fs. The red solid lines in panels (b) and (c) represent the best fits obtained. The dashed lines in panels (a) and (c) indicate the demagnetization times,τth, of about 100 fs. Figure 3 shows the magnetization ( M normalized to the unpumped magnetization, M 0 ) as a function of time delay for a series of increasing pump fluences. The solid lines reproduce fits by a double exponential expression (Equation (2)) to the data (triangles) based on a semi-empirical model (see Methods ), which allows us to extract parameters like the maximum demagnetization, the thermalization time ( τ th ) and the relaxation time from the spin degrees of freedom to others ( τ s−ph ) [20] . To obtain accurate values for τ s−ph , long-delay scans have been performed ( Fig. 3b ). The thermalization time can also be characterized [11] by the delay time τ M at which the drop in magnetization reaches 63% of its maximum. The values of τ th and τ M obtained for the different infrared pump fluence levels are summarized in Table 1 . The uncertainty on these values is lower than ±25fs ( Supplementary Table S1 ). One notes that the values of τ th are fluctuating within 10 fs around 100 fs with no clear fluence dependance. τ M appears also to be fluence independent and equal to 85 fs, although a slow increase with increasing fluence cannot be ruled out. A demagnetization of almost 45% ( Fig. 3c ) is achieved in the case of the highest fluence level used (11 mJ cm −2 ), which is just under the destruction threshold of the sample in our repetitive kilohertz experiment. Nevertheless, even for this rather high degree of demagnetization, compared with other studies, we do not observe an increase of the thermalization time. Figure 3: Magnetization as a function of time delay for the [Co−Pd]30 multilayer film. ( a ) Demagnetization curves obtained for different pump fluences: 4, 6, 7.5 and 9 mJ cm −2 (respectively; red, up; green, down; cyan, right; and purple, left triangles). The probe fluence, 5×10 −5 mJ cm −2 , is negligible compared with the pump fluence [26] . The solid lines represent the best fits obtained for each fluence. The characteristic thermalization times, τ th , found are all between 90 and 110 fs with an error of ±25 fs. No clear relation between the pump fluence and τ th has been observed. ( b ) Example of a long delay scan used to determine the spin-phonon relaxation constant, τ s−ph . Long delay scans have been performed for each fluence. ( c ) High-resolution demagnetization curve obtained for the highest possible pump fluence (11 mJ cm −2 ), yielding a demagnetization of 44% and clearly showing a thermalization time of ~100 fs. The red solid lines in panels ( b ) and ( c ) represent the best fits obtained. The dashed lines in panels ( a ) and ( c ) indicate the demagnetization times, τ th , of about 100 fs. Full size image Table 1 Maximum demagnetization and demagnetization times for increasing pump fluences. Full size table The observation of a short thermalization time, which in addition is independent of the degree of stimulated demagnetization, is rather surprising, considering the results of recent MOKE studies of ultrafast demagnetization in Co-based materials [11] , [30] . These studies have reported thermalization times ( τ M ) in the range of 150 to 300fs for demagnetization degrees from 15 to 50% ( Supplementary Fig. S4 ). Moreover, those results agree well with the electron—phonon-mediated spin-flip scattering model developed by Koopmans et al . for the description of the demagnetization process [11] . One might be tempted to explain this discrepancy by the presence of Pd in the sample. Indeed, the large spin–orbit coupling of Pd could enhance the spin-flip rate thus leading to a shorter thermalization time in our Co/Pd multilayer. This conclusion is, however, in contradiction with the results obtained by Boeglin and co-workers on a 15 nm thin Co 0.5 Pd 0.5 alloy film [20] saturated in an external magnetic field. Employing X-ray magnetic circular dichroism absorption spectroscopy in a transmission experiment, these authors determined an overall thermalization time, τ th , of about 280 fs, which is in close agreement with the MOKE results mentioned above. We note that X-ray magnetic circular dichroism originates from the same resonant magneto-optical effect as the contrast mechanism in our scattering experiment. Boeglin et al . [20] exploited ×it at the Co L 2,3 absorption edge, whereas the Co M 3 edge was used here. Furthermore, we can rule out the small structural difference between the alloy and our multilayer film as the origin of the difference in thermalization time. Indeed, the difference is minimal as the Co-layer thickness is only 0.4 nm. We confirmed this by repeating our experiment on such a CoPd alloy film (see ref. 26 for film details), which yielded an equally faster demagnetization time ( Fig. 4 ). 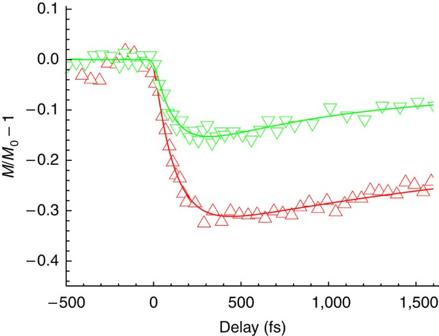Figure 4: Magnetization as function of time delay for the CoPd alloy film. Demagnetization curves obtained on a 50nm thin CoPd alloy film26for a pump fluence of 6 (green downward triangles) and 9mJ cm−2(red upward triangles). The solid lines represent the best fits. The corresponding parameters are reported inSupplementary Table S2. Figure 4: Magnetization as function of time delay for the CoPd alloy film. Demagnetization curves obtained on a 50nm thin CoPd alloy film [26] for a pump fluence of 6 (green downward triangles) and 9mJ cm −2 (red upward triangles). The solid lines represent the best fits. The corresponding parameters are reported in Supplementary Table S2 . Full size image To explain the faster demagnetization time observed here, four more experimental differences can be considered: the different probe photon energies used; the thickness of the magnetic layer; the presence or absence of an externally applied, static magnetic field; and the presence of a microscopic magnetic domain structure. The first point can be ruled out rather safely as it would be unreasonable to expect that the photon energies resonant with the Co M edge give shorter relaxation times than the both higher (Co L edge) and lower photon energies (infrared/visible; see Supplementary Fig. S4 ) [11] , [20] . We can equally rule out an effect of film thickness, since comparable thermalization times have been reported for Co-based films with thicknesses ranging from 15 to 110 nm [11] , [30] , [31] . The third point cannot be ruled out completely. We note, however, that MOKE studies have been performed in the presence and absence of an external magnetic field (in fact, complete time-resolved hysteresis loops were recorded [1] ) without revealing a difference in the thermalization time between these two modes. We are thus left with the last point, the presence of a nanometric magnetic domain structure in our experiment as origin of the observed faster thermalization time. This idea is supported by the recent publication of Malinowski et al . [8] These authors noticed that in a magnetic bilayer, spaced by a thin non-magnetic conductive layer, the demagnetization seems to be faster for an antiparallel orientation of the magnetization directions in the two layers. This led them to conclude that the laser-induced demagnetization process could be sped up by direct transfer of spin angular momentum between the two magnetic layers [8] . The magnetic domain structure of our sample can be seen as a network of such junctions. A direct transfer of spin angular momentum between neighbouring domains would then lead to an acceleration of the demagnetization process. We remark that the efficiency of this angular momentum transfer, and hence the magnitude of the demagnetization, depends on the number of excited carriers (hot electrons). The speed of the transfer, on the other hand, does primarily depend on the specific properties of the junctions. Thus, a thermalization time mostly independent of the degree of demagnetization would then be expected. The proposed mechanism is further supported by the theoretical work of Battiato et al . [12] , who show that spin-polarized transport of hot electrons from a magnetic layer to a metallic buffer may account for the early stage of ultrafast demagnetization. It seems natural to extend this theory to the case here, where transport would occur between neighbouring domains with opposite spin-polarization of their majority electrons. We note that, in comparison to typical velocities of hot electrons (up to 1nmfs−1 (ref. 12 )) the domain width (~80 nm) is reasonably small. After a few tens of femtoseconds, a significant exchange of spin-polarized electrons from neighbouring domains could have occurred, in line with our observation. We note that the proposed transport of spin-polarized electrons should induce changes in the domain walls between the neighbouring domains. Such changes could be resolved by recording higher diffraction orders or by direct time-resolved imaging of the magnetic domain structure, but neither was possible in the current experimental set-up. In summary, for the first time, laser-induced demagnetization was studied at the magnetic domain level with a time resolution of about 40 fs and a spatial resolution better than 100nm, thus exploiting the unique capabilities of soft X-ray HHG sources. It has been shown that magnetic domains exhibit locally a rapid loss of magnetization on the femtosecond timescale similar to the one observed in uniformly magnetized transition metal films studied so far. The magnetic domain structure itself remains mostly unaffected by the demagnetization process. A thermalization time of about 100 fs has been revealed, which is faster than has been reported previously [11] , [20] . In addition, we do not find any fluence level dependence of the demagnetization process for the range of 14 to 44% of total demagnetization. We provide evidence that the presence of the magnetic domain structure is potentially the origin of these observations via direct transfer of spin angular momentum between neighbouring domains. Sample preparation The sample is a [Co(0. 4 nm)/Pd(0.6 nm)] 30 multilayer deposited by magnetron sputtering on a 30-nm thin Si 3 N 4 multi-membranes (squares of 50×50 μm 2 ) chip. This multilayer exhibits an out-of-plane magnetic anisotropy. To enhance heat dissipation, a 30-nm thick Al buffer layer was used and to avoid oxidation a 2-nm thick Pd cap layer was added. The sample is demagnetized so as to present an aligned stripe domain state with an in-plane oscillating magnetic field [29] . Pump–probe experiment The pump–probe set-up is based on a Ti:sapphire laser ( λ 0 =815 nm), delivering 5 mJ, 40 fs (full-width at half-maximum (FWHM)), linearly polarized (horizontal) pulses at 1 kHz. Each pulse is split into a strong part and a weak part (pump) by a 90–10% beam splitter. The strong part is focussed into a gas cell filled with neon (35 mbar) to generate high harmonics (probe) by nonlinear interaction between the laser and the gas. The generated harmonics retain the polarization of the infrared laser and span a wide photon energy range between 40 and 78 eV (ref. 25 ). Tuning the source parameters allows optimizing the efficiency for the generation of the thirty-ninth harmonic, which matches the Co M 3 absorption edge located at 60 eV (ref. 26 ). To suppress the incident infrared light, a 200nm thick aluminum foil is introduced into the optical path. The transmitted harmonics are then focussed (focal spot of 30 μm in diameter) by a spherical mirror (focal length, 625 mm) coated with a wide-band-gap multilayer onto the sample. To select only the thirty-ninth harmonic, a second multilayer mirror, located a few centimetres before the sample, is used. The pump beam goes through a delay line (step size of 3 fs) and is focussed (focal spot of 150 μm in diameter) to excite the sample. The fluence of the pump beam can be adjusted and the size of the focal spot ensures an uniform illumination across one membrane. The harmonic light, elastically scattered by the magnetic domain structure of the sample, is collected by a PI-MTE CCD camera (Princeton Instrument) located 4 cm behind the sample and protected from any diffuse infrared light by an aluminum filter. This foil is supported by an Ni mesh that appears as a grid on the scattering patterns. The CCD pixels have been binned 4 by 4 yielding a pixel size of 54 μm. The time resolution of this experiment is less than 45 fs (FWHM), which is set predominantly by the infrared pulse duration (40 fs), because the harmonic pulses are much shorter [32] , [33] and because there is no jitter between infrared and harmonic pulses in this set-up. Data analysis Resonant magnetic scattering pattern were recorded for different time delays and pump fluences. These patterns are similar to what is expected from incoherent small angle X-ray scattering, although we are using a coherent X-ray beam. However, the speckles due to the coherence are too small to be observed because of the large illuminated area yielding incoherent-like scattering patterns. The charge scattering of diffuse X-rays, due to the square shape of the membrane, is partially blocked by the beam-stop and completely removed for data analysis. For radial integration of the scattering pattern, a recording time of 500 s was necessary whereas a 50s recording time was sufficient to obtain the demagnetization curves. The radial analysis was conducted by measuring the integrated intensity in ring with increasing radius, r , in pixels. Knowing the distance between the sample and the CCD camera, D =40 mm, the size of the pixels, 0.054 mm, and the wavelength of the light, λ =20.7 nm, the data were converted into wave-vector transfer, q , in nm−1, according to the following relation: The data were then fitted by a pseudo-Voigt profile (often used in X-ray scattering experiments). The demagnetization curves were obtained by summing the intensities of each pixel in the two scattering spots to obtain the integrated density that is proportional to the square of the magnetization (see below). Variations of the harmonic intensity yields a standard deviation of 2% for an integration time of 50 s. The data were then fitted by the following double exponential expression: where G ( t ) is the Gaussian function, H ( t ) is the Heavyside function and τ th and τ s−ph are, respectively, the thermalization time and the relaxation time from spins to other degrees of freedom [5] , [20] . This fit neglects the cooling down of the lattice system, which occurs on the nanosecond timescale and is thus of no relevance on the timescale studied here. Relation between magnetization and integrated intensity At a resonant energy, owing to magneto-optical effect, the magnetic domain structure can be approximated by a square grating whose transmission alternates between t + and t − for up-and-down magnetic domains. The diffracted intensity in the first order, I , of such a grating is given by [34] : where n ± , is the optical index of up (+) and down (−) magnetic domains [35] , d is the thickness of the film and, λ is the wavelength of the radiation. Developing expression 3, we find that I is proportional to where T is the average transmission of the grating. Given that Δ δ and Δ β are both proportional to the magnetization M (ref. 35 ), it follows: How to cite this article: Vodungbo, B. et al . Laser-induced ultrafast demagnetization in the presence of a nanoscale magnetic domain network. Nat. Commun. 3:999 doi: 10.1038/ncomms2007 (2012).